Host suppression of quorum sensing during catheter-associated urinary tract infections Chronic bacterial infections on medical devices, including catheter-associated urinary tract infections (CAUTI), are associated with bacterial biofilm communities that are refractory to antibiotic therapy and resistant to host immunity. Previously, we have shown that Pseudomonas aeruginosa can cause CAUTI by forming a device-associated biofilm that is independent of known biofilm exopolysaccharides. Here, we show by RNA-seq that host urine alters the transcriptome of P. aeruginosa by suppressing quorum sensing regulated genes. P. aeruginosa produces acyl homoserine lactones (AHLs) in the presence of urea, but cannot perceive AHLs. Repression of quorum sensing by urine implies that quorum sensing should be dispensable during infection of the urinary tract. Indeed, mutants defective in quorum sensing are able to colonize similarly to wild-type in a murine model of CAUTI. Quorum sensing-regulated processes in clinical isolates are also inhibited by urea. These data show that urea in urine is a natural anti-quorum sensing mechanism in mammals. Chronic bacterial infections on medical devices are associated with bacterial biofilm communities that are refractory to antibiotic therapy and resistant to host immunity [1] , [2] . Bacteria use quorum sensing to coordinate their behavior at high cell density to produce biofilm matrix components [3] , [4] , [5] . Quorum-sensing pathways from diverse Gram-positive and Gram-negative bacteria are required for infections in mammalian hosts [6] , [7] . Pseudomonas aeruginosa strain PAO1 defective in quorum sensing exhibited decreased biofilm formation in vitro [8] , [9] and reduced virulence in murine models of acute urinary tract infection [10] , [11] , acute pulmonary infection [12] , and burn wound infection [13] . Strategies to inactivate or interfere with quorum sensing have therefore been targeted in order to control bacterial infections [14] , [15] , [16] . Currently, the ability of mammalian hosts to interfere with bacterial quorum sensing is the subject of intense investigation [17] . Mammalian hosts encode paraoxonases, which are lactonases that can inactivate acyl homoserine lactone (AHL) and decrease P. aeruginosa biofilm formation, pyocyanin production, and protease activity in vitro [18] , [19] , [20] . However, the role of quorum sensing in chronic infections is not well understood. Here, we show that urea within host urine represses Pseudomonas aeruginosa quorum sensing in vitro and during catheter-associated urinary tract infections (CAUTI). Bacterial perception of homoserine lactone (HSL) quorum-sensing signals, 3-oxo-C 12 -HSL and C 4 -HSL, was disrupted, while ability to produce quorum molecules remained intact. These results imply that quorum sensing should be dispensable during infection of the urinary tract. This was tested by infecting quorum-sensing defective mutants of P. aeruginosa in a murine model of CAUTI. These mutants were able to colonize the catheter in a manner similar to wild type, indicating that quorum sensing is indeed dispensable during CAUTI. The contribution of quorum sensing was also assessed for human clinical CAUTI isolates. Quorum-sensing-regulated processes in a majority of human CAUTI isolates were inhibited by urea, while the remaining clinical isolates were found to be quorum defective, indicating that urine suppression of P. aeruginosa quorum sensing is a conserved process in mammalian systems. Overall, our data imply that urea in urine is a mammalian host factor that interferes with bacterial quorum sensing. RNA-seq reveals that urine and urea repress quorum sensing To investigate factors that are important during chronic infection, we established a murine model of CAUTI for the opportunistic pathogen P. aeruginosa . In this model, biofilm formation in the catheter lumen is dependent on extracellular DNA (eDNA) [21] , [22] and independent of the exopolysaccharides required for abiotic biofilms [23] , [24] . Murine urine and urea were able to induce these eDNA-dependent biofilms, indicating that P. aeruginosa specifically responds to urine and urea. To characterize this response, the transcriptome of P. aeruginosa grown in media supplemented with mouse urine, human urine or urea, or instilled into the mouse bladder, was assayed by RNA-seq. Bacteria exposed to mouse and human urine showed similar changes in gene expression (Fig. 1a and complete RNA-seq data are available in Supplementary Data 1 ), and an overlapping transcriptional response to urine, urea, and incubation within mice bladder was observed. A Venn diagram of genes that were ≥4-fold down-regulated in each condition (Fig. 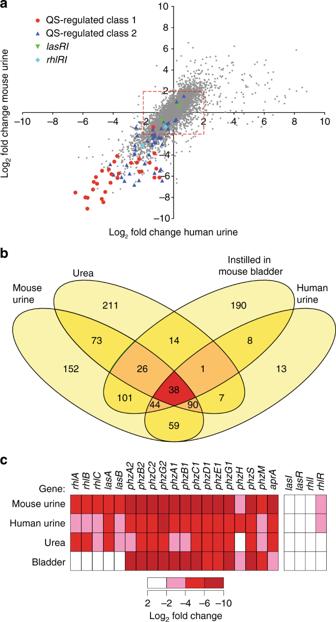Fig. 1 Urine and urea suppress the expression of quorum-regulated genes.aComparisons of log2fold changes in gene expression between LB vs mouse and human urine. Genes with less than four-fold change are within the box indicated by the red dashed line. The quorum-sensing-regulated genes were defined as those genes that had 20-fold decreased in Wagner et al.25and 40-fold decreased in Schuster et al.26in strains lackinglasI rhlIandlasR rhlR, respectively. Red circles indicate quorum-sensing-regulated genes that were identified in both studies (class 1), dark blue triangles indicate quorum-sensing-regulated genes that were identified in one of the two studies (class 2), green inverted triangles indicatelasRandlasIgenes, and light blue diamonds indicaterhlRandrhlIgenes.bVenn diagrams comparing the number ofP. aeruginosagenes with four-fold reduction in expression when grown in mouse urine, human urine, media containing urea, and instilled in the mouse bladder as compared to bacteria grown in LB.cHeat map showing log2fold gene expression changes of quorum-sensing-regulated genes in the presence of indicated urine, urea, and instillation into a mouse bladder 1b and Supplementary Table 1 ) shows that P. aeruginosa had a conserved response to mammalian urine and urea. Of note, aprA, rhlAB, rhlC , lasA , lasB genes, and phz operons, all genes known to be regulated by the las and rhl quorum-sensing systems, were among those most down-regulated in response to urea and urine (Fig. 1a, c ) [25] , [26] . Microarray studies have reported positive-feedback regulation of the lasI / lasR and rhlI / rhlR quorum regulatory systems [25] , [26] . This was also observed in our RNA-seq data, with lasI / lasR and rhlI / rhlR genes being down-regulated, albeit by less than four-fold, in response to urine, urea, or growth within the murine bladder (Fig. 1c ). Together, these results indicated that P. aeruginosa responds to growth in urine and media containing urea by altering its transcriptome in a manner similar to that of quorum-sensing mutants lacking AHL synthases or AHL receptors [25] , [26] . Fig. 1 Urine and urea suppress the expression of quorum-regulated genes. a Comparisons of log 2 fold changes in gene expression between LB vs mouse and human urine. Genes with less than four-fold change are within the box indicated by the red dashed line. The quorum-sensing-regulated genes were defined as those genes that had 20-fold decreased in Wagner et al. [25] and 40-fold decreased in Schuster et al. [26] in strains lacking lasI rhlI and lasR rhlR , respectively. Red circles indicate quorum-sensing-regulated genes that were identified in both studies (class 1), dark blue triangles indicate quorum-sensing-regulated genes that were identified in one of the two studies (class 2), green inverted triangles indicate lasR and lasI genes, and light blue diamonds indicate rhlR and rhlI genes. b Venn diagrams comparing the number of P. aeruginosa genes with four-fold reduction in expression when grown in mouse urine, human urine, media containing urea, and instilled in the mouse bladder as compared to bacteria grown in LB. c Heat map showing log 2 fold gene expression changes of quorum-sensing-regulated genes in the presence of indicated urine, urea, and instillation into a mouse bladder Full size image Urine and urea impair quorum-sensing-dependent phenotypes P. aeruginosa has several well-characterized quorum-regulated phenotypes, including elastase clearance on milk plates [27] , [28] , rhamnolipid production, and pyocyanin production [29] , [30] , [31] . We tested whether repression of quorum-regulated genes by urine and urea was significant enough to repress quorum-regulated phenotypes. Increasing amounts of mouse urine diminished elastase clearance zones on milk plates (Fig. 2a ), and decreased both rhamnolipid and pyocyanin production (Fig. 2b ). These phenotypes were not due to reduced growth, as P. aeruginosa grew to similar optical density in liquid cultures in the absence or presence of urine at the tested concentrations [21] . The concentration of urea in the pooled mouse and human urine was experimentally determined to be 786 ± 22 and 243 ± 14 mM, respectively. Addition of increasing concentrations of urea diminished elastase clearance zones on milk plates (Fig. 2c ) and further inhibited rhamnolipid and pyocyanin production (Fig. 2 d). The repression of quorum sensing by urine and urea was reversible as bacteria previously grown in media with 0.5 M urea were able to produce pyocyanin when subcultured in LB lacking urea (Fig. 2e ). Together, these results indicate that urine and physiological concentrations of urea can repress LasR- and RhlR-mediated quorum-regulated phenotypes. Fig. 2 Urine and urea suppress quorum-regulated phenotypes. P. aeruginosa grown in 1× phosphate-buffered saline + 1% tryptone (PBS-T) supplemented with increasing concentrations of human urine was quantified for a zone of clearance around bacterial colony grown on milk plates, b pyocyanin (red bars) and rhamnolipid (blue bars) production. P. aeruginosa grown in LB supplemented with increasing amounts of urea was quantified for c zone of clearance around colonies grown on milk plates, d pyocyanin (red bars) and rhamnolipid (blue bars) production. e Quantification of pyocyanin produced by P. aeruginosa after 24-h growth in the presence or absence of 0.5 M urea followed by 16-h subculture growth in the presence or absence of 0.5 M urea. Data represent the mean and standard deviation of at least three independent replicates and were analyzed by unpaired t -test using GraphPad Prism software. Asterisk (*, **, and ***) indicates p < 0.05, <0.01, and <0.001, respectively Full size image Urea impairs perception of 3-oxo-C 12 -HSL by P. aeruginosa Quorum sensing can be repressed either by inhibiting the production of AHLs or by preventing the perception of AHLs by their receptors. To determine if urea inhibited the production of AHLs, we used ethyl acetate to extract AHLs from spent media of P. aeruginosa strain PA14 grown in the presence or absence of urea. The extracts were assayed for the ability to restore quorum-sensing-dependent phenotypes in ∆ lasI or rhlI:Tn strains, which lack the respective synthases for 3-oxo-C 12 -HSL and C 4 -HSL quorum molecules. Extracts from PA14 grown either in the presence or in the absence of urea restored pyocyanin production in the rhlI::tn mutant similar to chemically synthesized C 4 -HSL (Fig. 3a ). Likewise, extracts from PA14 grown in the presence or absence of urea induced protease production from a ∆ lasI mutant similar to chemically synthesized 3-oxo-C 12 -HSL (Fig. 3b ). This extract-mediated induction was due to the presence of secreted AHLs, as extracts from the spent media of ∆ lasI did not induce protease activity by ∆ lasI (Fig. 3b ). While AHL concentration was lower when bacteria were grown in media containing urea, our data show that the levels of AHLs were above the threshold required to induce quorum sensing, suggesting that urea neither prevents secretion of quorum molecules nor chemically inactivates the quorum molecule. Fig. 3 Urea affects perception, but not production, of autoinducers. a Production of C 4 -HSL by P. aeruginosa grown in the presence and absence of urea was assessed by the ability of spent media extracts to promote production of pyocyanin by PA14, rhlI::Tn , and ∆rhlRI . b Production of 3-oxo-C 12 -HSL by P. aeruginosa grown in the presence and absence of urea was quantified by the ability of spent media extracts to promote protease activity by PA14, ∆lasI , and ∆lasR grown on milk plates. Extracts of culture supernatants from cells grown in the absence of urea (gray) and presence of urea (black) are indicated. c Perception of chemically synthesized C 4 -HSL (0.5 µM) as measured by pyocyanin production by PA14, rhlI::Tn , ∆rhlRI grown in LB in the absence and presence of 0.5 M urea. d Perception of chemically synthesized 3-oxo-C 12 -HSL (1 µM) as quantified by PA14, ∆ lasI, and ∆lasR grown on milk plates in the absence or presence of 0.5 M urea. Samples, in which control HSL was added, are indicated in red for C 4 -HSL and blue for 3-oxo-C 12 -HSL. e , f Beta-gal activity was measured for E. coli strain DH5α carrying either e pECP64 (ptac- lasR, lasB′-lacZ ) or f pECP61 (ptac- rhlR rhlA’-lacZ ) grown with 5 nM 3-oxo-C 12 -HSL or 5 µM C 4 -HSL, respectively, in the presence (solid) or absence (open) of 0.5 M urea. Data represent the mean and standard deviation of at least three independent samples for each incubation time. Data were analyzed by unpaired t -test using GraphPad Prism software. Asterisk (*, **, and ***) indicates p < 0.05, <0.01, and <0.001, respectively Full size image To determine if urea disrupts the perception of AHLs, chemically synthesized AHLs were added to wild type and synthase mutant bacteria in media with or without 0.5 M urea. In the absence of urea, the addition of C 4 -HSL restored pyocyanin production to a rhlI::tn mutant (Fig. 3c ) and addition of 3-oxo-C 12 -HSL restored elastase production in a ∆ lasI mutant (Fig. 3d ) to similar levels as observed for wild-type parental strains in the absence of urea. In contrast, the wild-type parental strain had significantly reduced pyocyanin and protease production in the presence of urea, and addition of excess AHLs failed to restore quorum-regulated responses. Likewise, the addition of C 4 -HSL or 3-oxo-C 12 -HSL to the respective synthase mutant strain failed to induce pyocyanin or elastase production in the presence of urea. Plasmid-derived over-expression of rhlR or lasR in the respective null mutants, while able to complement the respective mutations, did not overcome repression of quorum-regulated phenotypes by urea (Supplementary Figure 1 ). Since quorum regulation in P. aeruginosa is complex and involves many regulators, we asked whether urea repression of quorum sensing was also observed for lasR - and rhlR -regulated systems recapitulated in Escherichia coli [32] . E. coli strains expressing LasR can activate a lasB′-lacZ reporter when stimulated with exogenous 3-oxo-C 12 -HSL, but this activation was inhibited by the addition of 0.5 M urea (Fig. 3e ). Urea also inhibited the activation of a rhlA reporter by exogenously added C 4 -HSL in E. coli (Fig. 3f ), indicating that the process inhibited by urea is common to P. aeruginosa and E. coli . Together these results indicate that urea in urine disrupts quorum sensing by inhibiting bacterial perception of AHLs without chemically altering the AHL molecule. Urea does not prevent LasR-3-oxo-C 12 -HSL from binding to DNA Urea could inhibit AHL perception by either inhibiting the quorum receptor-AHL complex from binding to DNA or preventing the AHLs from activating the quorum receptor. To test whether urea inhibited the LasR-3-oxo-C 12 -HSL complex from binding DNA, purified recombinant LasR bound to 3-oxo-C 12 -HSL was assayed for DNA binding in the presence and absence of 0.5 M urea in vitro [33] , [34] . 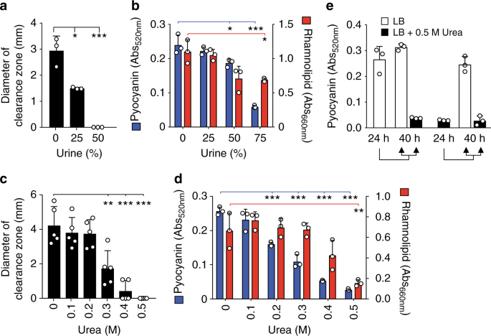Fig. 2 Urine and urea suppress quorum-regulated phenotypes.P. aeruginosagrown in 1× phosphate-buffered saline + 1% tryptone (PBS-T) supplemented with increasing concentrations of human urine was quantified forazone of clearance around bacterial colony grown on milk plates,bpyocyanin (red bars) and rhamnolipid (blue bars) production.P. aeruginosagrown in LB supplemented with increasing amounts of urea was quantified forczone of clearance around colonies grown on milk plates,dpyocyanin (red bars) and rhamnolipid (blue bars) production.eQuantification of pyocyanin produced byP. aeruginosaafter 24-h growth in the presence or absence of 0.5 M urea followed by 16-h subculture growth in the presence or absence of 0.5 M urea. Data represent the mean and standard deviation of at least three independent replicates and were analyzed by unpairedt-test using GraphPad Prism software. Asterisk (*, **, and ***) indicatesp< 0.05, <0.01, and <0.001, respectively The LasR-3-oxo-C 12 -HSL complex reduced the mobility of DNA fragments containing known las box but not control DNA sequences lacking las box (Supplementary Figure 2 ). The addition of urea did not alter the ability of this LasR-3-oxo-C 12 -HSL complex to bind DNA. Quorum-sensing genes are dispensable during CAUTI Based on the results showing urine inhibition of quorum sensing, we predicted that quorum sensing is not required to establish CAUTI and tested this hypothesis using a previously characterized murine model of CAUTI [21] , [35] . 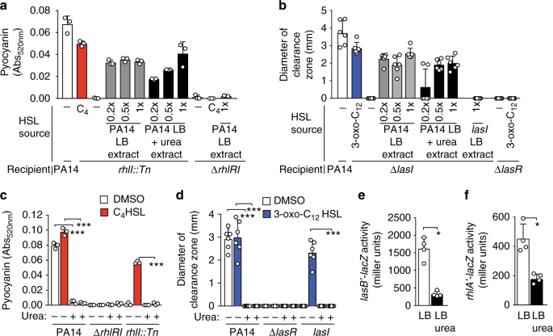Fig. 3 Urea affects perception, but not production, of autoinducers.aProduction of C4-HSL byP. aeruginosagrown in the presence and absence of urea was assessed by the ability of spent media extracts to promote production of pyocyanin by PA14,rhlI::Tn, and∆rhlRI.bProduction of 3-oxo-C12-HSL byP. aeruginosagrown in the presence and absence of urea was quantified by the ability of spent media extracts to promote protease activity by PA14,∆lasI, and∆lasRgrown on milk plates. Extracts of culture supernatants from cells grown in the absence of urea (gray) and presence of urea (black) are indicated.cPerception of chemically synthesized C4-HSL (0.5 µM) as measured by pyocyanin production by PA14,rhlI::Tn,∆rhlRIgrown in LB in the absence and presence of 0.5 M urea.dPerception of chemically synthesized 3-oxo-C12-HSL (1 µM) as quantified by PA14, ∆lasI,and∆lasRgrown on milk plates in the absence or presence of 0.5 M urea. Samples, in which control HSL was added, are indicated in red for C4-HSL and blue for 3-oxo-C12-HSL.e,fBeta-gal activity was measured forE. colistrain DH5α carrying eitherepECP64 (ptac-lasR, lasB′-lacZ) orfpECP61 (ptac-rhlR rhlA’-lacZ) grown with 5 nM 3-oxo-C12-HSL or 5 µM C4-HSL, respectively, in the presence (solid) or absence (open) of 0.5 M urea. Data represent the mean and standard deviation of at least three independent samples for each incubation time. Data were analyzed by unpairedt-test using GraphPad Prism software. Asterisk (*, **, and ***) indicatesp< 0.05, <0.01, and <0.001, respectively Bacterial persistence in this model results from catheter-associated colonization, as ≥10-fold higher numbers of bacteria were cultured from the catheter than from the bladder in 20 of 24 infected mice (Supplementary Figure 3 ). Mice infected with PA14 or the isogenic quorum-sensing mutants Δ lasR , Δ lasI , or Δ rhlRI had similar bacterial burdens in the bladder and kidneys, indicating that quorum sensing was dispensable for CAUTI (Fig. 4a ). Likewise, competitive infections with PA14 and Δ lasR or Δ rhlRI showed that both Δ lasR and Δ rhlRI were as likely to form biofilms on catheter and to establish chronic infection within the bladder as wild-type PA14 (Fig. 4b, c ). These results show that quorum sensing is not required for biofilm formation during CAUTI. Fig. 4 Quorum sensing is not required for catheter-associated urinary tract infection. a Bacterial load of the bladders and kidneys from mice infected with either PA14, ∆ lasR ,∆ lasI , or ∆ rhlRI using the CAUTI model of infection. The dashed line represents the limit of detection. Competitive indices (CI) for b biofilm formation in the catheter and c establishing infection in the bladder when mice were co-infected with PA14-lux and either unmarked PA14, ∆ lasR , or ∆ rhlRI in CAUTI. CI were calculated by first determining the ratio of lux+ and lux− CFU recovered from the catheter or infected bladder and then dividing by the ratio of lux+ and lux− CFU of the inoculum used for infection. Each symbol represents the CI measured for an individual bladder or a catheter. Dashed lines represent a CI value of 1 where no competition is observed. Horizontal line represents the geometric mean and error bars represent standard deviation Full size image If urine- and urea-mediated suppression of quorum sensing in P. aeruginosa also occurs during human CAUTI, we hypothesized that quorum sensing would be dispensable during human infections. To test this prediction, 29 clinical P. aeruginosa CAUTI isolates from human patients with urinary catheters or nephrostomy tubes were assessed for phenotypes that are indicative of quorum sensing [36] . 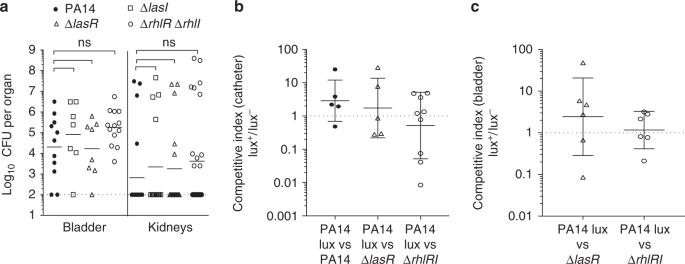Fig. 4 Quorum sensing is not required for catheter-associated urinary tract infection.aBacterial load of the bladders and kidneys from mice infected with either PA14, ∆lasR,∆lasI, or ∆rhlRIusing the CAUTI model of infection. The dashed line represents the limit of detection. Competitive indices (CI) forbbiofilm formation in the catheter andcestablishing infection in the bladder when mice were co-infected with PA14-lux and either unmarked PA14, ∆lasR, or ∆rhlRIin CAUTI. CI were calculated by first determining the ratio of lux+ and lux− CFU recovered from the catheter or infected bladder and then dividing by the ratio of lux+ and lux− CFU of the inoculum used for infection. Each symbol represents the CI measured for an individual bladder or a catheter. Dashed lines represent a CI value of 1 where no competition is observed. Horizontal line represents the geometric mean and error bars represent standard deviation 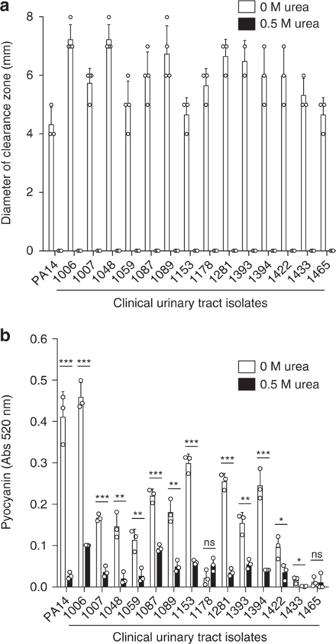Fig. 5 Urea suppresses quorum-sensing phenotypes inP. aeruginosaUTI clinical isolates.aDiameter of clearing around colonies for a selection ofP. aeruginosaUTI clinical isolates grown on milk plates supplemented with either no urea (white bars) or 0.5 M urea (black bars). Under these conditions, none of the clinical isolates had elastase activity when grown in media containing 0.5 M urea. All comparisons between no urea and 0.5 M urea have ap< 0.001.bUTI strains grown in the presence and absence of 0.5 M urea were assessed for pyocyanin production. Data represent the mean and standard deviation of at least three independent samples. Data were analyzed by unpairedt-test using GraphPad Prism software by comparing samples with no urea or 0.5 M urea. Asterisk (*, **, and ***) indicatesp< 0.05, 0.01, and <0.001, respectively and "ns" indicates not significant Fifteen of these 29 isolates did not swarm, exhibited no or minimal protease activity, and were scored as “quorum negative”; the other 14 were considered “quorum competent” based on their protease activity and ability to swarm [36] . For quorum-negative strains, sequencing of the lasRI and rhlRI genes revealed one isolate with an early stop codon in lasR at position 186, two isolates with an early stop codon in rhlR at positions 67 and 74, respectively, and an isolate where rhlR had a substitution of the conserved P56 to alanine (Supplementary Table 2 ). About 0.5 M urea repressed the protease activity of the 14 quorum competent clinical isolates (Fig. 5a ) and significantly reduced pyocyanin production in the 11 isolates that produced this phenazine (Fig. 5b ). The suppression of quorum-sensing-dependent phenotypes by urea in human CAUTI isolates, and the loss of lasR- and rhlR- dependent phenotypes in other human CAUTI isolates suggests that quorum sensing is indeed dispensable for CAUTI. In this setting, quorum-sensing receptors become dispensable during chronic CAUTI, allowing P. aeruginosa to accumulate mutations in quorum-sensing genes. Missense and nonsense mutations in the quorum-sensing receptor lasR are commonly observed in chronic isolates from the lungs of cystic fibrosis (CF) patients [37] , suggesting that quorum sensing may be dispensable during other P. aeruginosa chronic infections. Fig. 5 Urea suppresses quorum-sensing phenotypes in P. aeruginosa UTI clinical isolates. a Diameter of clearing around colonies for a selection of P. aeruginosa UTI clinical isolates grown on milk plates supplemented with either no urea (white bars) or 0.5 M urea (black bars). Under these conditions, none of the clinical isolates had elastase activity when grown in media containing 0.5 M urea. All comparisons between no urea and 0.5 M urea have a p < 0.001. b UTI strains grown in the presence and absence of 0.5 M urea were assessed for pyocyanin production. Data represent the mean and standard deviation of at least three independent samples. Data were analyzed by unpaired t -test using GraphPad Prism software by comparing samples with no urea or 0.5 M urea. Asterisk (*, **, and ***) indicates p < 0.05, 0.01, and <0.001, respectively and "ns" indicates not significant Full size image This study establishes that urea within urine is a host factor that inhibits expression of quorum-regulated genes in P. aeruginosa . Transcriptome analysis showed that P. aeruginosa responds to urea and urine by down-regulating genes that are involved in quorum sensing, while phenotypic assays showed that P. aeruginosa phenocopied a quorum-sensing null mutant in the presence of urine and urea. Thus urea acts as a natural inhibitor of quorum sensing in P. aeruginosa . Future studies will determine the mechanistic basis for urine/urea inhibition of quorum sensing. It is surprising that inhibition of AHL quorum sensing by urea or urine has not been previously reported, as urinary tract pathogens such as uropathogenic E. coli (UPEC), Enterobacter spp., Proteus mirabilis, and Klebsiella pneumoniae are well-studied [38] . Previous studies employing RNA-seq revealed the comprehensive transcriptome of UPEC isolates from human UTI patients [39] . E. coli is known to respond to AHL through the transcription factor SdiA [40] , a LuxR homolog [41] . Transcriptome analysis of these human UTI strains showed small (<4-fold) changes in expression levels of the SdiA regulon when UPEC isolates were grown in urine from healthy donors vs in LB media [39] . One reason for the absence of a urine-mediated effect on quorum-regulated genes in the UPEC study may be that enteric bacteria, such as UPEC, do not encode an endogenous AHL synthase gene [42] . The transcriptome study of UPEC isolates was performed in the absence of bacteria capable of producing AHLs that activate SdiA [39] . An effect of urea in urine on the SdiA regulon would not be expected in the absence of an exogenous source of AHL. Nonetheless, using the LasR system reconstituted in E. coli , we observed that growth in media containing urea reduced the expression of a lasB -lacZ reporter gene [31] . Future studies will determine if urine/urea inhibition of bacterial quorum sensing is a general process that affects all AHL utilizing systems and other bacterial quorum molecules such as autoinducer-2 and autoinducing peptides. [6] , [43] During infection of mammalian host, quorum sensing is critical for acute infections of the lung [12] , urinary tract [10] , [11] and burn wounds [44] by P. aeruginosa . The role of quorum sensing during chronic infection by P. aeruginosa is still under active investigation. One of the key lines of evidence implicating quorum sensing in chronic P. aeruginosa infections comes from studies of CF isolates [37] , [45] , [46] . Sequencing of longitudinal strains from the same CF patient revealed that P. aeruginosa could cause a life-long infection and, during this prolonged infection, accumulate mutations in mutS , mucA , and lasR among many other genes [37] , [47] , [48] . Null mutations in mutS are found in 35–50% of CF isolates, explaining the often observed hypermutability of CF isolates [47] , [49] . Mutations in mucA leads to derepression of the AlgU/AlgT sigma factor resulting in the constitutive expression of the alginate biosynthesis ( algD-A ) operon [50] , [51] . As a consequence, these strains have increased production of the alginate exopolysaccharide [52] , which leads to reduced lung function of CF patients. While the effects of mutations in mutS and mucA on P. aeruginosa CF isolates have been well characterized, the effect of mutations in lasR is still debated. One hypothesis of why lasR function is lost during chronic lung infection is that lasR mutation provides an adaptive growth advantage in the low nutrient environment of the CF lung [45] , [53] . An alternative hypothesis posits that lasR mutants are social cheaters that benefit from quorum-sensing-regulated proteins made by neighboring bacteria without paying the metabolic cost of contributing to their production [54] . We would like to propose a third hypothesis in which the high frequency of lasR mutations present in clinical P. aeruginosa isolates reflects the absence of a requirement for quorum sensing during chronic infection. Similar to chronic CF isolates, P. aeruginosa isolates from human patients with CAUTI have acquired mutations in lasR and display null lasR quorum-sensing phenotypes. In murine chronic CAUTI infections, we have shown that quorum sensing is in fact dispensable as quorum-sensing null mutants successfully competed with wild-type P. aeruginosa in establishing chronic infection. The differences in the requirement of virulence factors between acute infections and chronic infections should change our view of chronic infections and lead to the development of treatment strategies that are specific for chronic infections. Bacterial cultures and growth conditions rhlR , rhlI , and lasI transposon mutants were obtained from the P. aeruginosa PA14 non-redundant transposon insertion mutant library provided by the Ausubel Lab at Harvard Medical School, Boston, MA [55] . In-frame deletion mutants and HA-tagged genes were made using primers listed (Supplementary Table 3 ). For in-frame deletion mutants, 1 kb regions upstream and downstream of the gene were cloned into pCR-Blunt. Then the two 1 kb fragments were subcloned into a pEX vector [56] . The in-frame deletion was introduced into wild-type P. aeruginosa PA14 by conjugation of the pEX deletion plasmid using the E. coli HB101 pRK2013 helper strain. Unmarked in-frame deletion mutations were selected by sucrose counter-selection, screened by PCR and confirmed by sequencing. Complementation strains were made by cloning the genes into pCR-Blunt vector and then transferring the gene to a pMMB expression vector. The E. coli strains expressing the plasmids were then mated with the corresponding P. aeruginosa knockout strain. All strains were grown in either LB or 1× PBS + 1% tryptone (PBS-T). Collection of human and mouse urine Urine was collected from human volunteers with informed consent in accordance with the Institutional Review Board at the University of Maryland, College Park. Identifying information about the volunteers were not collected at the time of sample donation. Urine was sterile filtered through a 0.2 µm filter, pooled, and stored at −80 °C until use. Mouse urine was collected from anesthetized mice by insertion of sterile catheter tubing. Urine was collected from the catheter, pooled, sterile filtered, and stored at −80 °C until use. RNA sequencing library preparation and analysis RNA was isolated from bacteria grown in LB, LB + 0.5 M urea, PBS-T, PBS-T + 75% human urine, or PBS-T + 75% mouse urine using Qiagen RNeasy Mini Kit (cat no. 74104). For the in vivo RNA-seq, P. aeruginosa was instilled into bladders of anesthetized mice for 90 min prior to collection and RNA isolation. Ribosomal RNA was removed from total RNA using the Epicentre Ribo-Zero Magnetic Kit (cat no. MRZGN126). Ribosomal-free RNA was then fragmented and cDNA library was prepared using Epicentre ScriptSeq v2 RNA-Seq Library Preparation Kit (cat no. SSV21106). RNA-seq libraries were sequenced using Illumina HiSeq 1000 at the Institute for Bioscience & Biotechnology Research (IBBR) at University of Maryland, College Park. Sequences were aligned to the PA14 reference genome using Bowtie2 (ref. [57] ). Interactive Genome Viewer was used to visualize the data. Fold changes were determined using DESeq. Quantification of pyocyanin Pyocyanin was quantified using a spectrophometric method [58] . Indicated P. aeruginosa strains were grown in LB for 16 h while shaking at 37 °C. Overnight cultures were then diluted 1:1000 in LB supplemented with either 0, 0.1, 0.2, 0.3, 0.4, or 0.5 M urea or PBS-T supplemented with 25%, 50%, or 75% human urine and subcultured for an additional 16 h at 37 °C. Following subculturing, the optical density (OD 600 ) was measured. Cultures were centrifuged at 16,100 g for 5 min. The supernatant (1.25 ml) was then extracted with 500 µl chloroform. Pyocyanin-containing chloroform extracts were extracted again with 250 µl 0.2 N HCl, which protonates pyocyanin changing the color from blue to red. Pyocyanin was quantified by measuring absorbance ( A 520 ) in a spectrophotometer [58] . When testing for reversibility of quorum phenotypes, pyocyanin was quantified for the overnight cultures grown in LB with or without 0.5 M urea. Each of the overnight cultures were then used for 1:1000 subcultures in media with or without 0.5 M urea. After an additional 16 h, pyocyanin was assayed. Protease assay Protease activity was assessed using milk agar medium [59] . Overnight cultures of indicated P. aeruginosa strains were diluted to approximately 5 × 10 4 bacteria per ml. One microliter of the diluted culture was spotted on the surface of protease agar plates containing 2% (w/v) nutrient agar and 2.5% (w/v) non-fat dried milk and supplemented with indicated amounts of urea or human urine. Protease agar plates were incubated at 37 °C for 16 h or just before protease activity was detected from the negative control ∆ lasI . Pictures of plates were taken using a Fuji LAS3000 Imager and zone of clearance was determined by subtracting the diameter of colonies from the diameter of clearing using ImageJ software. Rhamnolipid assay Rhamnolipids were quantified using a colorimetric assay [60] . A volume of 4 ml of supernatant was isolated from 5 ml of overnight P. aeruginosa cultures. Rhamnolipids were extracted from supernatants using equal volumes of ethyl acetate. The ethyl acetate layer was transferred to a new tube and the extraction was repeated three times. The ethyl acetate extractions were combined and evaporated. The remaining precipitant was then resuspended in 4 ml chloroform and 400 µl methylene blue solution, mixed vigorously, and then allowed to incubate at room temperature for 15 min to allow for color development. One milliliter of the methylene blue/chloroform layer was transferred to a clean 2 ml microfuge tube and 500 µl of 0.2 N HCl was added. When mixed with acid, the methylene blue in the chloroform layer shifts from a blue to a red color in the aqueous layer. Rhamnolipids are quantified by transferring 200 µl of the aqueous layer to a flat bottom 96-well plate and measuring the absorbance at 660 nm using a spectrophotometer. Urea assay Urea was quantified using a colormetric method by measuring the absorption of the dye dimethylaminobenzaldehyde (DMAB) (see Method 967.07 in Official Method of Analysis by ACOC [61] ). A volume of 100 µl of 0.1 M DMAB was added to 100 µl of standard concentrations (0, 5, 10, 25, 50, and 100 mM) of urea resuspended in artificial urine media. Standards were thoroughly mixed and allowed to incubate at room temperature for at least 5 min and absorbance was measured at 420 nm. Quantification of urea present in human and mouse urine samples was analyzed simultaneously with standards. Dilutions were made of the urine in order for absorbance to be read within range of the standard curve and the spectrophotometer. Effect of urea on rhl and las systems expressed in E. coli Bioassays to test the activity of AHLs in E. coli were performed using a modified procedure [31] . Overnight cultures of E. coli strain DH5α carrying either pECP64 or pECP61.5 were diluted into fresh supplemented A medium [62] to an OD 600 of 0.1 and incubated with shaking at 37 °C until OD 600 of 0.5. While E. coli were growing, assay tubes were prepared with AHL by drying under N 2 . After addition of IPTG to a final concentration of 1 mM to the E. coli cultures, 950 μl aliquots of cultures were transferred to tubes that contained each AHL with indicated concentrations of urea. Cultures in tubes were incubated at 37 °C with shaking for 90 min after which β-galactosidase (β-gal) activity was measured using the Miller assay [63] . Extraction of autoinducers Cultures of wild-type PA14 or ∆ lasI were grown shaking overnight at 37 °C in 100 ml LB or LB + 0.5 M urea. Prior to centrifugation, aliquots of the overnight culture were removed to measure OD 600 and colony-forming units (CFU). The supernatants of overnight cultures were collected and extracted twice with 90 ml acidified ethyl acetate using a separating funnel. Ethyl acetate extracts were then dried and resuspended in a calculated volume of DMSO that allows for normalization of bacterial CFU. Chemically synthesized C 4 -HSL (#10007898) and 3-oxo-C 12 -HSL (#10007895) were purchased from Cayman Chemical. Murine CAUTI All studies and procedures were approved by the University of Maryland Institutional Animal Care and Use Committee (IACUC) and complied with all relevant ethical regulations. Murine infections were performed using CF-1 mice [21] . Mice were injected with 1.5 × 10 7 CFU P. aeruginosa strain transurethrally after a 5-mm catheter was inserted in the bladder of anesthetized mice. Bladders and kidneys were harvested 1–2 weeks post infection. Only mice whose bladders still retained the 5 mm catheter at the end of the experiment were considered. For some experiments, catheters were removed from the bladders by extrusion through the urethra. Bacterial burdens were determined by first homogenizing catheter, bladder, or each kidney in 1 ml sterile 1× PBS-T followed by plating serial dilutions on LB agar plates to determine CFU.